Frequency domain optical parametric amplification Today’s ultrafast lasers operate at the physical limits of optical materials to reach extreme performances. Amplification of single-cycle laser pulses with their corresponding octave-spanning spectra still remains a formidable challenge since the universal dilemma of gain narrowing sets limits for both real level pumped amplifiers as well as parametric amplifiers. We demonstrate that employing parametric amplification in the frequency domain rather than in time domain opens up new design opportunities for ultrafast laser science, with the potential to generate single-cycle multi-terawatt pulses. Fundamental restrictions arising from phase mismatch and damage threshold of nonlinear laser crystals are not only circumvented but also exploited to produce a synergy between increased seed spectrum and increased pump energy. This concept was successfully demonstrated by generating carrier envelope phase stable, 1.43 mJ two-cycle pulses at 1.8 μm wavelength. In electrical engineering, function generators are used to test the response function of electronic circuits down to the nanosecond time scale. To test the ‘response function’ of bound electrons in atoms or molecules on the attosecond (1 asec=10 −18 s) time scale, optical function generators have been developed [1] , [2] , [3] . Rather than modifying only the intensity profile of an ultra short laser pulse, these devices tailor the electric field oscillations within the pulse’s intensity envelope. Such intracycle shaping of laser waveforms is an extremely powerful tool as strong field phenomena are driven by the field gradient rather than the cycle-averaged intensity envelope [4] , [5] . Inevitably, these devices are spectrally extremely broadband (exceeding one octave), yet their pulse energy is limited to a few nJ up to 300 μJ. As in electronics, further amplification is desirable for intracycle controlled light fields. Historically, the breakthrough in ultrafast high-power laser science came with chirped pulse amplification (CPA) in 1985.It enabled lowering the peak power during amplification by temporally stretching the pulses [6] . CPA systems, however, lack the capability of few-cycle operation as the gain of the amplifying medium is not constant across the pulse spectrum. This reduces the spectral bandwidth during amplification, generally referred to as gain narrowing. Therefore, the most widespread scheme to generate intense few-cycle pulses thus far relies on external compression in a hollow-core fibre subsequent to the actual laser amplifier [3] , [7] , which is limited to a few mJ [8] . In 1992, the CPA concept was extended to optical parametric chirped pulse amplification (OPCPA) [9] , which enabled true high-power amplification of mJ level, sub-three-cycle pulses [10] , [11] , [12] , [13] , [14] , [15] . Nevertheless, satisfying the phase-matching condition over an optical octave, along with the crystal damage thresholds still denote fundamental limitations in the design of OPCPA. Coherent combination of different OPCPA’s has been demonstrated [1] , [2] , [16] at the expense of increased complexity. In this paper, we present a different strategy for high-power parametric amplification of carrier envelope phase (CEP) stable pulses that overcomes fundamental material limitations (gain bandwidth, damage threshold) and offers new design opportunities. As opposed to traditional schemes where laser pulses are amplified in the time domain, we propose to amplify their corresponding spectral parts independent of each other in a frequency domain optical parametric amplifier (FOPA). In this manner, simultaneous upscaling of pulse energy and amplified bandwidth becomes possible. This single device paves the way for amplification of subcycle pulses without increasing their duration. It can also be beneficial for future multicycle ultrahigh-energy systems where damage threshold of laser crystals and large compression gratings are an issue. The concept of FOPA At the core of FOPA is the strategy of amplifying a very broad spectrum ‘slice by slice’ by distributing its frequencies ω over different crystals in the Fourier plane (FP) as depicted in Fig. 1 . This enables amplification without phase-matching limitations because the total gain bandwidth is now given by the number of crystals employed and not by the optical properties of each crystal. The same argument holds regarding material damage thresholds as the Fourier transformation of time domain pulses spreads out their spectrum onto a spatial coordinate along the x -axis as well. The correct spectral slicing is provided in a 4-f setup [17] that performs an optical Fourier transformation before and after amplification. This arrangement inherently stretches few-cycle input pulses to picosecond (1 ps=10 −12 s) durations in each focal spot in the FP and recompresses them afterwards without a dedicated stretcher–compressor arrangement. 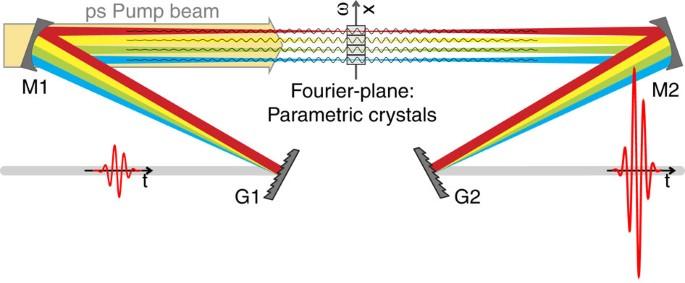Figure 1: The concept of frequency domain optical parametric amplification. Transform-limited input pulses are spectrally dispersed in a symmetric4-fsetup and remain transform limited leaving the FOPA without the requirement for a stretcher–compressor stage. Ultra broadband phase matching is achieved by spreading the spectrum over many (four in our case) individually tunable, nonlinear crystals, and thus is not limited by the properties of a single crystal. At the same time, this spreading distributes incident energies over a large area with the consequence that an increased seed spectrum or energy can be amplified by increasing the number of crystals, eliminating restrictions imposed by limited crystal apertures. As the effective pulse duration in each focal spot in the Fourier plane is in the picosecond range, the FOPA is pumped by picosecond pulses, which further increases the damage threshold. Figure 1: The concept of frequency domain optical parametric amplification. Transform-limited input pulses are spectrally dispersed in a symmetric 4-f setup and remain transform limited leaving the FOPA without the requirement for a stretcher–compressor stage. Ultra broadband phase matching is achieved by spreading the spectrum over many (four in our case) individually tunable, nonlinear crystals, and thus is not limited by the properties of a single crystal. At the same time, this spreading distributes incident energies over a large area with the consequence that an increased seed spectrum or energy can be amplified by increasing the number of crystals, eliminating restrictions imposed by limited crystal apertures. As the effective pulse duration in each focal spot in the Fourier plane is in the picosecond range, the FOPA is pumped by picosecond pulses, which further increases the damage threshold. Full size image Traditionally, CPA and OPCPA systems amplify different colours of a temporally stretched pulse in a time sequential manner, making it difficult to tackle gain narrowing. Gain narrowing mainly occurs because of (i) limited gain bandwidth in CPA, (ii) increasing phase mismatch in long parametric crystals and (iii) the temporal intensity envelope of the pump beam in OPCPAs. All these limitations are circumvented by FOPA. Fourier domain amplification has been performed experimentally by other groups [18] , [19] , [20] , [21] , [22] . However, only multicycle pulses with sub-mJ pulse energies have been demonstrated (except ref. 21 for 70fs pulses). Compared with previous experiments, FOPA offers two crucial differences that enables single-cycle pulse amplification: (i) the application of parametric crystals instead of real level gain media and (ii) the use of more than one crystal in the FP. Employing a parametric process rather than a population inverted gain medium largely relaxes issues stemming from heat deposition. Therefore, FOPA neither distorts the spatial beam profile nor adds an uncompensated spectral phase, because thermal-lensing effects are absent [20] , [22] . Furthermore, distributing an octave of frequencies over more than one crystal has many advantages, as will be discussed below. To date, amplification of the shortest sub-two-cycle, mJ-level pulses has been demonstrated only in the IR region when the pump wavelength is close to the ‘magic wavelength’ (wavelength where the group delay dispersion (GDD) for signal and idler vanishes around degeneracy) [11] , [13] . FOPA can be performed throughout the entire transmission range of nonlinear crystals as long as pump lasers are available. Experimental realization of FOPA The FOPA was designed as an upgrade to the existing CEP stabilized two-cycle IR beam line at the Advanced Laser Light Source (ALLS) described in the methods section and in refs 23 , 24 . These pulses are used to seed the FOPA with 200 μJ of pulse energy. The core of the FOPA is a 4-f setup shown in Fig. 1 explained in more detail in the Methods section and supplementary Fig. 1 . When both gratings are placed at the focal distance from the collimating mirrors (M1 & M2) and the mirror distance is 2f , the setup is referred to as symmetric 4-f setup, which does not introduce any change to the input temporal pulse shape at the exit. After spectrally dispersing the input beam on grating G1 and collimation with M1, each wavelength is focused to a 200 μm spot size in the FP. This spot size in combination with grating dispersion and focal length of M1 define the seed pulse duration in the FP, which is about 1.4ps as explained in the Methods section and supplementary Fig. 2 . The FP contains four identical type I BBO crystals. Each crystal aperture is 4 × 15 mm with the long side oriented parallel to the horizontally dispersed spectrum in the FP. Thus, four crystals side by side cover the spread spectrum extending over 60 mm in the FP. It is emphasized that parametric amplification of a sub-two-cycle bandwidth does not require four different BBO crystals as the phase-matching angle varies very slowly for the given conditions (see supplementary Fig. 3 ). The motivation to employ multiple crystals was to demonstrate the scaling capabilities of the FOPA concept. Synchronization of the four different wavelength channels was accomplished by polishing all four crystals in one batch to ensure their same relative optical thickness as is discussed in the Methods section. After the FP, an identical mirror-grating arrangement performs a second Fourier transformation to recover the time domain pulses with the same pulse duration as at the input. Finally, we draw attention to the peculiarities of the pump beam. The task is to provide a uniform intensity distribution along the horizontal axis in the FP, that is, the axis of the spread spectrum. Simple beam expansion of Gaussian beams in the horizontal direction combined with focusing in the vertical direction using cylindrical optics still provides a Gaussian intensity distribution along the FP. To modify this intensity distribution, we employed a special aspheric lens (‘Powell lens’) that spreads out the light rays stronger at the centre while containing them more at the edges, which leads to an intensity enhancement at the edges [25] , see supplementary Figs 4 and 5 for more details. Our current design offers ~10% higher pump intensity in the spectral wings than in the centre. Thus, a suitably designed pump beam path not only serves to pump the parametric process but it also enables tailoring the gain function across the spectrum by enhancing the intensity at the outer parts in the FP. Characterization of spectral, temporal and spatial beam properties First, we discuss the spatial and spectral properties of the FOPA output, followed by its temporal performance. A typical broadband seed spectrum of a two-cycle pulse ranging from 1.4–2.2 μm is given by the red line of Fig. 2a . The spectral range incident on each of the four crystals is marked by numbers 1–4. The transmitted spectrum (shaded grey) is two times magnified and shows no significant spectral reshaping after the FOPA. Small spectral discontinuities are evident at positions marked by the vertical lines, which represent a joint between two neighbouring crystals. The absence of pronounced dips indicates negligible effects imposed by the sharp crystal edges in the FP. The overall transmission is 48% yielding an output energy of 100 μJ. 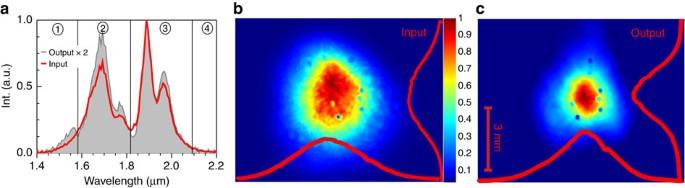Figure 2: Characteristics of the output beam. (a) Comparing the spectral transmission of the unamplified output beam (shaded grey curve) to the input spectrum (red curve) shows no significant spectral reshaping effect of FOPA. The total transmission is 48%. (b) Spatial beam shape of the seed beam after the hollow-core fibre and (c) after maximum amplification subsequent to the FOPA. The small spots across the beam profile arise from dust on the CCD camera. Figure 2b shows the seed beam profile after the hollow-core fibre which was recorded with a two-photon process on a standard CCD camera (more details are given in the Methods section). Figure 2: Characteristics of the output beam. ( a ) Comparing the spectral transmission of the unamplified output beam (shaded grey curve) to the input spectrum (red curve) shows no significant spectral reshaping effect of FOPA. The total transmission is 48%. ( b ) Spatial beam shape of the seed beam after the hollow-core fibre and ( c ) after maximum amplification subsequent to the FOPA. The small spots across the beam profile arise from dust on the CCD camera. Full size image When pumping the FP with 12.8 mJ,~2ps pulses at a centre wavelength of 800 nm, an energy of 1.76 mJ was measured in the FP. This corresponds to an output energy of 1.43 mJ due to the 75% transmission of one half of the 4-f setup. The energy stability was <3% rms and the corresponding beam profile is shown in Fig. 2c . The dependence of the amplified pulse energy on the pump energy is shown in Fig. 3b by the black line. Throughout the available pumping range in the FP from 2.9 mJ up to 12.8 mJ, this dependence stays linear without showing saturation. Likewise, the conversion efficiency stays at a constantly high level of ~14% (red curve in Fig. 3b ), which is higher than previously reported for IR OPCPAs [11] , [13] . Remarkably, no superfluorescence is observed when blocking the seed beam at maximum pump level. 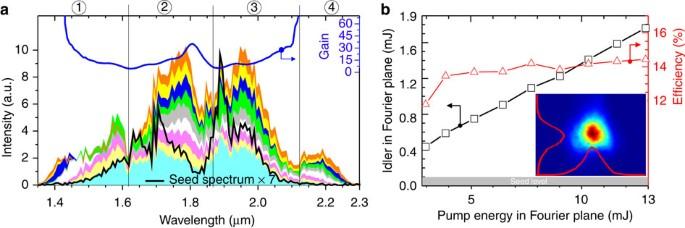Figure 3: Characteristics of the amplified beam. (a) Spectral characterization subsequent to the FOPA. The magnified seed spectrum (after broadening in a hollow-core fibre) of the sub-2 cycle pulse is displayed as the black curve. Individual spectral ranges of the four type I BBO crystals (1–4) employed in the Fourier plane are marked by thin vertical lines. The coloured spectra recorded for different pump levels exhibit no spectral narrowing up to the maximum level (orange curve). The experimentally obtained gain curve (blue) shows an increase towards the outer spectral parts underlining the gain tailoring opportunity of the FOPA. (b) The linear dependence of amplified idler energy versus pump energy in the Fourier plane shows no saturation and a constantly high efficiency of about 14%. The inset shows the spatial beam profile of the 1.4 mJ output pulses. Figure 3: Characteristics of the amplified beam. ( a ) Spectral characterization subsequent to the FOPA. The magnified seed spectrum (after broadening in a hollow-core fibre) of the sub-2 cycle pulse is displayed as the black curve. Individual spectral ranges of the four type I BBO crystals (1–4) employed in the Fourier plane are marked by thin vertical lines. The coloured spectra recorded for different pump levels exhibit no spectral narrowing up to the maximum level (orange curve). The experimentally obtained gain curve (blue) shows an increase towards the outer spectral parts underlining the gain tailoring opportunity of the FOPA. ( b ) The linear dependence of amplified idler energy versus pump energy in the Fourier plane shows no saturation and a constantly high efficiency of about 14%. The inset shows the spatial beam profile of the 1.4 mJ output pulses. Full size image To demonstrate the minor influence of pump beam impurities on the amplified beam, we reduced the pump power by 50% and scanned an Allen key across the pump beam. As amplification takes place in the FP, no change of spatial quality was observed at the FOPA output, only a homogenous intensity decrease. We also characterized the spatial chirp, that is, the variation of the spectrum along the horizontal or vertical direction of the beam profile shown in Fig. 2c . No spatial chirp was observed neither for the unamplified FOPA output nor the case of maximum amplification as is shown by supplementary Fig. 6 . The next step was to investigate the dependence of gain bandwidth on amplification. The results are presented in Fig. 3a . The coloured curves correspond to a successively increased pump energy in steps of 10% (starting at 20% of maximum) according to the data points of Fig. 3b . Strikingly, the broad seed bandwidth from 1.35 μm up to 2.25 μm remains at all amplification levels. The spectral wings are even favoured relative to the intense central part. This behaviour is clearly reflected in the spectral gain curve (blue line in Fig. 3a ), which shows higher gain for the spectral wings. The gain curve is obtained by dividing the amplified by the seed spectrum. Temporal characterization of the seed, FOPA transmitted, and FOPA amplified pulses was performed using second harmonic generation-frequency resolved optical gating (SHG-FROG) [26] . 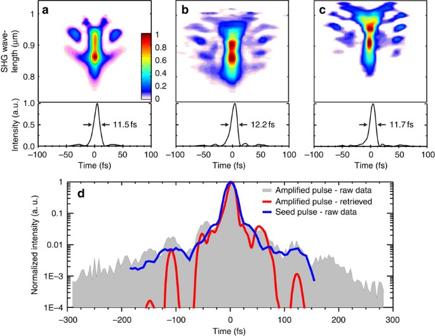Figure 4: Temporal characterization with SHG-FROG. Figures (a–c) display the measured spectrograms in the upper row and the retrieved temporal intensity below. The lowest contour line corresponds to values around 1% of the peak in the spectrogram. (a) Shows the seed pulses whereby a duration of 11.5 fs at a center wavelength of 1.8 μm denotes 1.9 optical cycles at full width half maximum of intensity. (b) The clean temporal profile of the seed pulses remains after passing through the FOPA. (c) At maximum output energy of 1.43 mJ, the pulse shape shows no degradation effects after 15-fold amplification. (d) Evaluation of pulse contrast and SHG-FROG retrieval quality on a logarithmic scale. The plots for the raw data are obtained by projecting the 2D spectrogram onto the time axis. Several pedestals of the amplified pulse shown as shaded grey become apparent (3–5% level around ±50 fs; 1% level around ±110 fs; per mille level around ±160 fs). Remarkably, the pedestal structure of the retrieved sub-2-cycle pulses (red curve) agrees with the raw data down to the 1% level 100 fs away from the main peak. Pedestals on the per mille level are not retrieved. By comparing the raw data of seed and amplified pulses, one recognizes that the pedestals around ±100 fs are already present in the seed itself. A slight increase around +50 fs is seen which, however, does not affect the total energy contained in the main pulse within ±50 fs. An in depth characterization of the SHG-FROG performance is given bysupplementary Figs 7–11. Figure 4 shows measured SHG-FROG traces (values between 1–6% of the peak in the spectrogram are highlighted in magenta, while values below 1% appear as white colour) in the upper part and the retrieved temporal intensity profile underneath. A relatively clean sub-2-cycle pulse with small pedestals, shown in Fig. 4a , was used to seed the FOPA. Eighty-five per cent of the total energy is contained in the main pulse. This good temporal contrast remains unchanged after passing through the FOPA with the pump beam blocked, as can be seen in Fig. 4b , which means that the sharp crystal edges in the FP do not introduce additional pedestals visible on a linear scale. At maximum amplification to 1.43 mJ, the FWHM duration still remains below two-cycles ( Fig. 4c ) with a slightly extended pedestal structure whereby the main pulse still contains 88% of the total energy or 105 MW pulse energy, respectively. This temporal contrast behaviour is further discussed by aid of the logarithmic plots in Fig. 4d comparing the raw autocorrelation data of the seed pulse (blue curve) with the one for the amplified pulse (shaded grey). Amplified pulses were scanned over ±300 fs, while the seed pulses were scanned over ±200 fs. Obviously, the 1% pedestals around ±110 fs are already present in the seed pulses. The lower dynamic range of the seed pulses prevented examination beyond 200 fs of time delay. A slight reduction of pulse contrast at the 3–5% level around ±50 fs is observed after amplification. Still, the current result of 1.9 cycle pulses clearly surpasses the best result achieved with a spectrally dispersed Ti:Sa amplification scheme [21] by a factor of two in terms of pulse energy and a factor of three in terms of number of cycles. Figure 4d furthermore underlines the quality of our FROG retrieval (red line), which is able to retrieve the pedestal structure on the 1% level. The typical FROG error is about 2 × 10 −3 for a grid size of 256 × 256. For a comprehensive analysis of the SHG-FROG retrieval together with a full presentation of raw data the reader is referred to supplementary Figs 7–11 . Figure 4: Temporal characterization with SHG-FROG. Figures ( a – c ) display the measured spectrograms in the upper row and the retrieved temporal intensity below. The lowest contour line corresponds to values around 1% of the peak in the spectrogram. ( a ) Shows the seed pulses whereby a duration of 11.5 fs at a center wavelength of 1.8 μm denotes 1.9 optical cycles at full width half maximum of intensity. ( b ) The clean temporal profile of the seed pulses remains after passing through the FOPA. ( c ) At maximum output energy of 1.43 mJ, the pulse shape shows no degradation effects after 15-fold amplification. ( d ) Evaluation of pulse contrast and SHG-FROG retrieval quality on a logarithmic scale. The plots for the raw data are obtained by projecting the 2D spectrogram onto the time axis. Several pedestals of the amplified pulse shown as shaded grey become apparent (3–5% level around ±50 fs; 1% level around ±110 fs; per mille level around ±160 fs). Remarkably, the pedestal structure of the retrieved sub-2-cycle pulses (red curve) agrees with the raw data down to the 1% level 100 fs away from the main peak. Pedestals on the per mille level are not retrieved. By comparing the raw data of seed and amplified pulses, one recognizes that the pedestals around ±100 fs are already present in the seed itself. A slight increase around +50 fs is seen which, however, does not affect the total energy contained in the main pulse within ±50 fs. An in depth characterization of the SHG-FROG performance is given by supplementary Figs 7–11 . Full size image Finally, a very important laser parameter for strong field physics driven by high-energy few-cycle pulses is the CEP. Thus, confirmation that FOPA preserves the CEP during amplification is very important. The f-2f measurement is shown in Fig. 5 . The stability was recorded for 1.7 min, each measurement denoting an average over 10 laser shots. Before the FOPA, the rms value was evaluated to be 320 mrad, which increased to 460 mrad after amplification as shown by the plot for the relative phase change in the lower panel of Fig. 5 . The increased CEP fluctuations might be caused by the fact that different Ti:Sa compressors are used for pumping the OPA prior to the hollow-core fibre and the FOPA itself, which introduces timing jitter and pointing fluctuations since a difference in optical beam path of about 10 m has to be balanced. 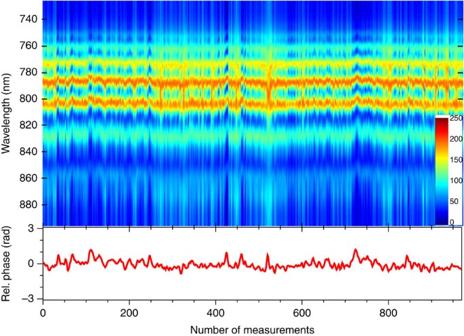Figure 5: Passive carrier envelop phase stabilization. The upper panel shows the evolution of the interference fringes in anf-2finterferometer over a period of 100 s. The system is free running, that is, without any feedback loop to correct for CEP fluctuations and each measurement is averaged over 10 laser shots. The relative phase is evaluated to be 460 mrad (lower panel). The stability of the input pulses delivered by the hollow-core fibre compressor is about 320 mrad. Figure 5: Passive carrier envelop phase stabilization. The upper panel shows the evolution of the interference fringes in an f-2f interferometer over a period of 100 s. The system is free running, that is, without any feedback loop to correct for CEP fluctuations and each measurement is averaged over 10 laser shots. The relative phase is evaluated to be 460 mrad (lower panel). The stability of the input pulses delivered by the hollow-core fibre compressor is about 320 mrad. Full size image Several individually tunable crystals in the FP allow the FOPA to function like multiple coherently combined narrow band OPAs. Each of them is free of phase-matching constrains due to the reduced bandwidth of about 200 nm for each crystal. However, this spectral slice of about 200 nm impinging on each crystal does not define the seed pulse duration in the FP. Instead, it is defined by the focal spot size in the FP in combination with the dispersion of the grating, as discussed in the Methods section. In the FP, the seed pulse duration becomes a function of the input beam diameter and the grating dispersion. Durations from 1 to 30 ps can be easily designed, meaning that conditions comparable to conventional OPCPAs can be met in the FP. Thus, all advantages known from OPCPA apply here as well, but FOPA offers many additional benefits. Note that in each focal spot in the FP, the ps pulses are transform limited (TL) unlike in OPCPA where the temporal gain curve can narrow the temporally chirped seed spectrum. We will briefly outline further benefits as they will become important for future expansions of the FOPA concept. As seen from the layout in Fig. 1 , in contrast to time domain amplification schemes, no additional stretcher–compressor arrangement is needed. If the FOPA is seeded with weak TL seed pulses, the amplified output pulses are already compressed. Nevertheless, it can also be seeded with chirped pulses. Furthermore, unlike previous sub-2 cycle OPCPAs, the whole setup does not require a pulse-shaping device to compress the laser output close to its TL pulse duration. This reduces cost, complexity and optical losses. Another favourable aspect is the absence of superfluorescence background in the output beam [11] necessary to achieve good ps pulse contrast. Ultimately, a major advantage of our scheme is the scalability of pulse energy and bandwidth at the same time. If the FOPA is seeded with an increased bandwidth, the spectrum in the FP will expand further and one simply has to add more crystals to amplify the entire spectrum. As the total area in the FP becomes larger, more pump energy can be delivered for amplification. In turn, to increase the pump energy for a constant seed bandwidth, one has two options. First, the FP can be enlarged by using either a grating with higher groove density or a collimating mirror with longer focal length. Second, the spherical mirror (M1) that focuses each colour into a radial spot in the FP can be replaced by a cylindrical mirror to increase the total amplification area by orders of magnitude. The key point is that by employing FOPA, the available aperture size of nonlinear crystals is no longer a limiting factor [13] as one can simply increase the number of (small aperture) crystals. Thus, we propose to implement FOPA to generate single-cycle multi-terawatt laser pulses. Although introduced in the framework of few-cycle pulses, FOPA can also be beneficial for multicycle petawatt systems offering the advantage that only one small grating is necessary for temporal recompression in contrast to the current state of the art where huge compressor chambers with multiple gratings are needed. As mentioned earlier, all sub-2-cycle IR OPCPAs operate around the degeneracy wavelength to achieve broadband phase matching. In contrast, FOPA can be used throughout the entire spectral transmission range of nonlinear crystals and one could even combine different crystal materials in the FP to enhance the transmission range and efficiency. One could also combine multiple pump beams at different wavelengths obtained from high average power ps laser systems. In this regard, the limitation is given by the availability of pump lasers. One concern that could be raised is the influence of the sharp crystal edges in the FP. Do these sharp edges corrupt the output beam either spatially or temporally? The answer is no, because the fundamental properties of optical Fourier transformation prevent spatial structures in the frequency domain from being transferred into spatial changes of the output beam. The practical consequence is that requirements on spatial pump beam quality are relaxed as impurities of the pump beam will not be transferred to the amplified beam. On the basis of simulations presented in the supplementary Fig. 12 , we see the temporal effect of sharp spectral edges to give rise to a ps contrast of 10 −5 and a nanosecond contrast better 10 −9 . This contrast can be enhanced by reducing the number of crystals and will eventually not be a limitation anymore if only one crystal is used. Another aspect is the thermal load at high average powers [27] which, in addition to spatial beam distortions, may cause undesirable variations of the spectral phase necessitating the use of an adaptive pulse-shaping device for compensation. On the other hand, as thermal load stems from absorption at the crystals transmission edges, one could, in principle, minimize such issues by combining different nonlinear materials in the FP. Regarding other limitations of the FOPA concept, the main bottleneck, apart from providing sufficient pump energy, is the beam recombination on the exit grating. Considering a damage threshold of 0.25 J cm −2 Horiba web page: http://www.horiba.com/scientific/products/diffraction-gratings/ (2013)., 10 TW single-cycle pulses are feasible with a beam diameter of 18 mm (1/e2 of intensity). Besides the damage threshold, the maximum spectral bandwidth supported at high efficiency can become an issue when aiming for octave-exceeding amplification [28] , [29] , [30] , [31] . The currently used grating exhibits good transmission from 1.1–2.5 μm, which supports subcycle pulse durations. In conclusion, by implementing Fourier domain optical parametric amplification, we have introduced a concept that turns the tables on a general dilemma in ultrafast laser amplifiers. The usual trade off between large bandwidth and high energy no longer holds and these two parameters can be increased simultaneously, in principle exceeding one octave of bandwidth at the multi terawatt level and beyond (see discussion below). Our first proof-of-concept demonstration yielded record-breaking performance in the field of few-cycle IR lasers: 1.43 mJ, two-cycle pulses (0.12TW) at 1.8 μm wavelength with a CEP stability of 460 mrad. Amplified CEP-stable single-cycle pulses will pave the route from the observation of asec ionization dynamics towards asec control experiments. The availability of high energy two-cycle laser pulses will enable the generation of high peak power asec pulses enabling: table-top X-ray nonlinear optics, XUV pump–XUV probe experiments, table-top X-ray imaging or the seeding of free electron lasers up to keV photon energy range, to name a few examples. Laser system The laser system used for the generation and amplification of few-cycle IR pulses was a 25 mJ, 45fs, 100 Hz Ti:Sa laser (Thales) from which 5 mJ were used to pump a white light-seeded OPA (HE-TOPAS, Light Conversion). The OPA delivers passively CEP stabilized idler pulses of 50 fs duration at 1.8 μm wavelength, which are compressed to two-cycle duration by nonlinear propagation in a hollow-core fibre followed by subsequent compression with bulk material [23] . In particular, this scheme relies on the combined action of self-steepening during nonlinear propagation in the fibre whose induced spectral phase asymmetry largely cancels the negative second order dispersion of FS in the anomalous dispersion regime at 1.8 mm together with its higher order dispersion terms. In this manner, 200 μJ seed pulses were coupled to the FOPA. The FOPA was pumped by the remaining 20 mJ, which are stretched to roughly 2 ps duration with a separate grating compressor. The overall transmission of the pump line from the compressor to the FP was about 66%. The Powell lens to generate the line focus of the pump beam was designed and fabricated by Osela Inc. FOPA details The dispersion gratings G1 and G2 for the FOPA setup shown in Fig. 1 have a groove density of 75 lines per mm with a blaze angle of 3.6° (Newport). The collimating mirrors M1 and M2 have a focal length of 800 mm giving rise to a spectral spread of about 60 mm in the FP. We now turn the attention to discuss details for planning a FOPA setup in which different constraints partially depend on each other Constraint no. 1: the overall geometrical arrangement. A more detailed scheme of the FOPA that is shown in the supplementary Fig. 1 . These aspects are important as there is a coupling between different parameters relevant for parametric amplification (seed focal spot size, pulse duration, intensity, bandwidth incident on each crystal, total expansion of the FP). Before describing these details, we discuss general aspects on building a zero dispersion 4f setup that preserves sub-2-cycle pulse duration. The beam path of Fig. 1 in the main paper is extended by more details in the supplementary Fig. 1 restricted to a single wavelength for reasons of clarity. In practice, each wavelength of the broadband pulse follows its specific optical path causing all different wavelength spots to be focused next to each other on a line along the FP. In a perfectly symmetric 4f setup (grating, collimating optic and FP are separated from each other by one focal length), the FP is a plane of symmetry. However, small displacements of the exit grating in the mm range as indicated in supplementary Fig. 1 can be used to precompensate small amounts of dispersion stemming from vacuum chamber windows, and so on. This octave-spanning variable chirp compensation is another advantage of the FOPA. For small displacements between 1 mm and 5 mm (sufficient to compensate up to 5 mm of FS), no spatial chirp of the output beam was observed. To minimize the effects of higher order chirp, the gratings are used under Littrow condition: α=β=ε, with α being the incident angle, β, the reflected angle and ε, the blaze angle of the grating. Furthermore, spherical aberrations from both mirrors would reduce the spatial beam quality and result in an uncompensated spectral phase as well, distorting the two-cycle pulse temporal profile. Therefore, the incident angle γ was set close to zero and a long focal length f of 800 mm was chosen. Next, we discuss specific constraints when aiming to operate FOPA in the sub-2-cycle regime. While phase matching of sub-2 cycle pulses can be reached with less than four crystals for the given combination of pump and seed wavelengths, the use of four crystals is motivated to prove the extension capabilities of FOPA. We chose to distribute this bandwidth over four BBO crystals. A crystal size of 15 mm (width) × 4 mm (high) × 4 mm (thickness) was chosen because a crystal dimension of 15 mm is available at low cost. Thus, the total expansion in FP is 4 × 15 mm=60 mm. The total expansion of the FP is a trade off between being large enough to conveniently handle multiple crystals next to each other and being small enough to allow using standard optical components (all optics used in the FOPA setup are ≤3″ diameter). Constraint no. 2: the choice of the diffraction grating. Its selection criteria include: right groove density, g, to achieve the correct spectral spread in the FP (generally in favour of low-groove densities to enable using long focal length mirrors), and a constantly high diffraction efficiency over the targeted spectral range without too much spectral modulation. The groove density influences the total expansion in the FP (see constraint no. 1) and the pulse duration in the FP. The later is because each focal spot of supplementary Fig. 1 in the FP is given by the diffraction limit of the optic used, that is, it has a finite size d f . This finite spot size contains a certain spectral bandwidth depending on the dispersion of the grating. Pulse durations from 1 to 30 ps can be achieved in the FP depending on the overall design of the setup. However, the pulse duration in the FP is largely independent on the input pulse duration; it is mainly defined by the geometrical optical properties of the 4f setup, as will be described in constraint no. 4. We like to point out that the ps pulses in each focal spot are not chirped but transform limited. This is another advantage of FOPA over OPCPA where the temporal chirp of seed pulses causes a loss of spectral bandwidth when overlaid with the temporal gain profile of the pump pulse. Constraint no. 3: the focusing optic. As mentioned before, a long focal length f is desirable to minimize spherical aberrations. The focal length (= mirror distance from the grating) together with the groove density g ( constraint no. 2) defines the total expansion in the FP ( constraint no. 1). It also influences the spot size d f (see constraint no. 4) and hence the seed pulse intensity in the FP. Unlike previous work on OPCPA where the seed and pump foci were unmatched to reduce super fluorescence generation [32] , we aimed to match the focal spot sizes of seed and pump beams in the FP to maximize conversion efficiency and gain. Constraint no. 4: the input beam diameter d in . It defines the spot size d f of each wavelength in the FP and can be used to adjust the pulse duration because the focus diameter sets the effective bandwidth in the FP. Thus, the pulse duration is inversely proportional to the input diameter. On the other hand, the intensity in a laser focus in principle increases proportional to the square of the input beam diameter. For the FOPA, the situation differs as an increased input beam diameter simultaneously reduces pulse duration (~d in ) and reduces focal area (~d in 2 ). Thus, the intensity in the FP increases only linearly with the input beam diameter. Finally, the input beam diameter equals the output diameter and thereby defines the fluence on the exit grating after amplification which should be kept below the damage threshold. To find the global design optimum of this multi dimensional parameter space, the FOPA was modelled numerically. Supplementary Fig. 2 shows the spectral spread in the FP for a bandwidth from 1.3–2.3 μm as a contour plot for a combination of different grating groove densities and focal lengths. The intersection point marked by dashed lines corresponds to a spot size of 210 μm associated to a seed pulse duration of about 1.4ps. A total spectral spread of about 55 mm in the FP is also convenient to realize the whole setup with 3″ optics. The total area in the FP is 55 mm × 0.2 mm equal to 0.1 cm 2 . Phase-matching conditions We chose to distribute an 800 nm bandwidth over four type I BBO crystals such that each crystal deals with an incident bandwidth of about 200 nm. Type I phase matching was chosen due to its broader phase-matching bandwidth compared with type II and its slightly higher effective nonlinearity. We point out that this total bandwidth could be easily phase matched with less than four crystals. Using four crystals, one can, in principle, extend the current setup to phase match more than one octave of frequencies. Single-cycle pulses, however, are not yet available with the laser system used. Supplementary Fig. 3 shows the phase-matching angle (θ) versus wavelength for a pump wavelength of 800 nm. To tune a type I BBO over the total spectral range, maximum 0.6° angle tuning is necessary. This small-angle tuning range relates to the fact that the degeneracy point at 1.6 μm falls within the tuning range. If the FOPA would be realized far away from the degeneracy wavelength of the pump beam, one might have to use four crystals cut at different phase-matching angle to phase match an entire octave. Due to this small-tuning range required, we decided to buy four identical crystals (United Crystals, the production tolerances are 0.1–0.2°) and to tune each crystal by ±0.2°, which does not affecting the overall transmission. The four identical type I BBO crystals in the FP were cut at θ=20.8 ° . The clear aperture of each crystal is 4 × 15 mm that expands the total spectral spread of about 55 mm across the four crystals. The thickness of 4 mm enables phase matching a 250–300 nm FWHM bandwidth over the entire tuning range. The collinear seed and pump beams are incident at a small angle of about 3° with respect to the normal of the BBO crystals. As this offset is the same for all crystals, it does not affect the relative timing. Small BBO angle tuning of ±0.2° allows phase shifting for about 1 μm of optical beam path. From the crystal back reflection, we estimated a required tuning range of smaller than 0.1° to bring all four channels in phase. This optimization was done looking at the shortness of the SHG autocorrelation to maintain two-cycle duration. In other words, the BBO crystals are used to amplify their corresponding spectral slices and to ensure fine phase adjustments on the order of the wavelength between the different channels. No active stabilization between the four channels is required since all are reflected off the same optics. We also performed an independent measurement of the relative crystal thickness using a conventional light microscope with NA of 0.75 and visible light (<1 μm resolution). Because the image size of 0.5 × 0.6 mm is much smaller than the BBO size of 4 mm, we used a high precision translation stage (<1 μm resolution) to scan the crystal length under the microscope objective. For each scan, we placed two crystals side by side to measure their absolute and relative thickness. The absolute thickness of the crystals is 4.056 mm. The relative thickness varies between 1.3 μm and 1.7 μm. The uncertainty of this measurement is 1.5 μm. This proves that the variation between different crystals is on the order of (or less than) the wavelength of 1.8 μm, which can be easily compensated by tilting the crystals as described above. Spatial beam-intensity profile : The intensity profile of the IR laser beams with a centre wavelength of 1.8 μm (corresponding to a photon energy of 0.67 eV) was characterized with a conventional Si based CCD camera. Although the Si band gap of 1.11 eV prohibits detection of lower energetic photons, with fs laser pulses a two photon process ca be excited in the Si detector [33] . In this case, the measured beam profile deviates from the real intensity distribution due to the higher order process. The measured profile appears narrower. Therefore, we characterized the photon order of the process in the Si by recording images as a function of input pulse energy. A near quadratic behaviour was found (factor 1.87). Thus, we deconvolved the measured intensity profile assuming a second order process, i.e. by multiplying the data with the square root of 2. Pulse characterization Temporal characterization of the 1.8 μm pulses was carried out with a home built SHG-FROG. It features geometrical beam splitting with a half mirror to ensure an all reflective setup. The use of a thin type I BBO crystal of 10 μm thickness in which beams are focused under a small angle enables measurement of sub-2 cycle pulses. As pulse retrieval in the sub-2 cycle regime requires a lot of care to be taken, we refer the interested reader to the book by Rick Trebino [26] and the corresponding chapters therein which describes all the steps that we took into account here as well. To cross check the quality of the retrieval, one can compare the retrieved temporal intensity with the experimental autocorrelation as is shown in Fig. 4d . The position of pedestals down to a 1% value of the peak maximum is retrieved correctly. Another cross check is the comparison of the retrieved spectrum with the independently measured one which is shown in supplementary Fig. 5 . A further comparison between raw data, data used for the retrieval input and retrieved FROG traces is provided in supplementary Figs 9–11 . An NIR spectrometer (Ocean Optics) is used to measure the IR spectrum from 1.3–2.3 μm. CEP stability was confirmed with an inline f-2f interferometer comprising a variable attenuator, white light generation in a FS plate, second harmonic generation of the IR spectrum in a type I BBO and a polarizer to project both the white light spectrum and its doubled fundamental on a common axis. About 3.5% of the beam was sent to the f-2f interferometer, while the measurement was carried out at a FOPA output energy of 0.7 mJ to avoid material damage. The evaluated CEP error after the FOPA amounts to 460 mrad rms while the rms after the hollow-core fibre was about 320 mrad. We believe that the 320 mrad after the fibre already reflect the noisy environmental conditions present in the laboratory. Another source for measuring an increased fluctuation after the FOPA might be the f-2f setup itself. Generally, we found it very hard to find proper conditions to generate a stable white light with the 2 cycle pulses either after the fibre or the FOPA. Picosecond pulse contrast behaviour As the sensitivity of our SHG autocorrelation was limited to about 10 −3 , we performed numerical simulations of the sharp crystal edges to give a rough picture of their influence. Supplementary Fig. 12a shows a Gaussian spectrum corresponding to a two-cycle pulse around 1.8 μm. The blue curve shows an unperturbed spectrum, while the red curves exhibits quiet pronounced gaps, which are positioned not symmetrically like is the case in the experimental setup. The limited resolution of our NIR spectrometer prevents us from resolving the experimental gap and the width shown clearly denotes an upper limit. Supplementary Fig. 12b ) plots the Fourier transformation of both curves showing two different regions: 500 fs around the main peak a fs contrast ratio better 10 −3 is visible, while this contrast improves towards the ps time scale to a ratio better than 10 −5 . At one nanosecond the contrast is about 10 −9 (data not shown). These theoretical contrast values improve by more than one order of magnitude if three crystals are used instead of four (data not shown). Further enhancement can be achieved by reducing the number of crystals in the FP. We used four crystals for the two-cycle pulses to underline the scalability towards multiple crystals in the FP. Clearly, three crystals are sufficient to phase match one octave of bandwidth. And with three crystals, the contrast at 4ps in Supplementary Fig. 9 reduces from 10 −5 to 10 −6 (10 −11 ns contrast). Subsequent contrast enhanced is possible by using plasma mirrors, which typically show 80% efficiency and 2–3 orders of magnitude contrast enhancement. Pump beam delivery Seed and pump beam travel collinearly in the FP and are combined with dichroic beam splitters before the FP and separated afterwards. Neither one of the pulse fronts is tilted. As mentioned in the main paper, expanding a Gaussian pump beam with standard spherical cylindrical optics would result in a Gaussian intensity distribution along the FP, that is, along the spread spectrum causing the outer spectral wings to experience much less gain than the central part, as depicted supplementary Fig. 4a . On the other hand, to make full advantage of the new design possibilities with the FOPA, one can modify the pump intensity distribution arbitrarily to match a desired gain function across the spectrum. We implemented a specially designed aspherical lens (Powell lens, Osela Inc.) in combination with a standard spherical optic for collimation to generate an intensity distribution which is slightly enhanced (10% with respect to the centre) towards the outer part of the FP as shown in supplementary Fig. 4b in the lower part. Supplementary Fig. 5 presents a 6 mm cut along the pump beam intensity distribution showing a merely constant behaviour with a slight increase towards the outer side (left side in Figure b). Supplementary Fig. 5c shows transverse cuts of the intensity distribution. The seed beam (220 μ) is about 25% smaller than the pump beam of 300 mm. Future scalability As mentioned, in the current setup, the total area in the FP covered by seed and pump, respectively, is about 55 mm × 0.2 mm equal to 0.1 cm 2 . This area can be upscaled by using cylindrical collimating mirrors instead of the spherical ones used here. In this way, the clear aperture can be extended to the full height dimension of each crystal. Damage threshold of BBO is in the range of 10 GW cm −2 for 100 ps pulses ( http://www.u-oplaz.com/crystals/crystals02.htm ), which corresponds to 1 J cm −2 . Standard BBO crystals dimensions nowadays exceed 20 × 20 mm clear aperture. Using five BBOs, with a clear aperture of 2 × 2 cm, gives a total area for pumping of 20 cm 2 . Pumping at 0.5 J cm −2 (half the damage threshold) over an area of 20 cm 2 denotes total pump energy of 10 J. Assuming moderate 10% conversion efficiency shows that Joule level, single-cycle pulses are feasible with FOPA (0.17PW). On the basis of those estimations, we are convinced that the FOPA is the most promising approach to bring single-cycle pulses to the sub-Petawatt level. How to cite this article: Schmidt, B. E. et al. Frequency domain optical parametric amplification. Nat. Commun. 5:3643 doi: 10.1038/ncomms4643 (2014).